Microtubule disruption synergizes with oncolytic virotherapy by inhibiting interferon translation and potentiating bystander killing In this study, we show that several microtubule-destabilizing agents used for decades for treatment of cancer and other diseases also sensitize cancer cells to oncolytic rhabdoviruses and improve therapeutic outcomes in resistant murine cancer models. Drug-induced microtubule destabilization leads to superior viral spread in cancer cells by disrupting type I IFN mRNA translation, leading to decreased IFN protein expression and secretion. Furthermore, microtubule-destabilizing agents specifically promote cancer cell death following stimulation by a subset of infection-induced cytokines, thereby increasing viral bystander effects. This study reveals a previously unappreciated role for microtubule structures in the regulation of the innate cellular antiviral response and demonstrates that unexpected combinations of approved chemotherapeutics and biological agents can lead to improved therapeutic outcomes. Oncolytic viruses (OVs) are self-amplifying cancer biotherapeutics that destroy malignancies without harming normal tissues. Derived from a variety of viral species, OVs are often engineered to exploit well-known hallmarks of cancer, including deregulated metabolism and proliferation, evasion of cell death and inefficient antiviral signalling [1] . Within the tumour, these agents destroy the malignancy by inducing direct oncolysis, stimulating antitumour immune responses and promoting tumour-vasculature shutdown (reviewed in ref. 2 ). While promising early- and late-phase clinical trials employing OVs to treat cancers continue to generate great enthusiasm, heterogeneity in clinical response remains a challenge [2] , [3] , [4] . To this end, it has been long recognized that improvements to therapeutic efficacy either through viral engineering or through combination therapies will be critical to the success of these platforms [2] , [5] . Rhabdoviruses such as vesicular stomatitis virus (VSV) have been used preclinically as a backbone to generate OVs for over a decade [6] , [7] , [8] and are now beginning clinical evaluation (for example, NCT01628640). While wild-type rhabdoviruses such as VSV (wtVSV) preferentially replicate in cancer cells, their tumour selectivity can be greatly improved through genetic engineering, for example, by capitalizing on the frequently defective capacity of tumours to engage antiviral programmes [6] , [7] , [8] . One of the first characterized and widely studied oncolytic strains of VSV (VSVΔ51) harbours a deletion at methionine 51 in the matrix (M) protein, blocking its ability to interact with nuclear pore proteins and prevent the export of cellular antiviral mRNAs from the nucleus to the cytoplasm [9] . As a result, VSVΔ51 cannot replicate in normal cells that have fully functional antiviral systems but replicates robustly in tumour cells that have lost the ability to mount an effective antiviral response. Capitalizing on cancer-specific defects in cellular immunity makes for remarkably safe and selective therapeutics; however, this can come at a significant cost in terms of efficacy. While VSVΔ51 can cure animals of some tumours incapable of producing or responding to interferon (IFN), nearly a third of cancer cell lines are essentially normal in this capacity, severely limiting viral spread and oncolysis [6] . Several genetic approaches have been explored and can be effective to overcome this roadblock. This includes using more potent viral backbones [8] , [10] , or expressing therapeutic transgenes to impair the IFN response [11] . Enhancing potency through genetic modification, nonetheless, carries some levels of risk and could compromise the excellent safety record OVs have enjoyed to date [2] . We have explored the concept of ‘conditionally enhancing’ OV growth and replication by transiently complementing genetically attenuated OVs using pharmacological agents. For example in earlier work, we have shown that treatment of resistant tumour cells with histone deacetylase (HDAC) inhibitors that downregulate IFN-responsive genes [12] leads to increased oncolysis by VSVΔ51 (ref. 13 ). More recently, we screened a small molecule library to discover novel enhancers of VSVΔ51-mediated oncolysis and identified distinct chemical entities that unexpectedly share the common feature of destabilizing microtubules. We report here a previously unappreciated role of microtubule structures in the control of type I IFN translation and show that microtubule-destabilizing agents (MDAs) specifically enhance the growth and spread of oncolytic rhabdoviruses in cancer cells and sensitize uninfected tumour cells to cytokine-mediated cell killing. MDAs enhance cancer-specific viral oncolysis A high-throughput screening approach [14] identified seven approved drugs that have microtubule-destabilizing activity among 15 previously unknown compounds found to enhance VSVΔ51-mediated oncolysis. 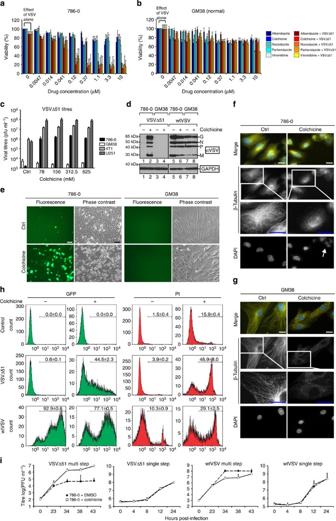Figure 1: MDAs enhance VSVΔ51 spread in cancer but not normal cells. (a,b) 786-0 cancer (a) and GM-38 normal (b) cells were pretreated with MDAs (xaxis) and then challenged with VSVΔ51, MOI 0.01. Forty-eight hours later, cell viability was assessed. (c) 786-0, U251 and 4T1 cancer cells as well as GM-38 were pretreated with colchicine (xaxis) and infected as above for 48 h and supernatants titred. (d,e) 786-0 and GM-38 cells were treated with 100 nM colchicine or vehicle before infection with VSVΔ51-GFP or wtVSV, as above. At 48 h post infection, phase contrast and fluorescent images were taken (e, scale bar, 50 μm), and cell lysates subject to western blot, where VSV proteins are indicated by arrows (d). (f,g) 786-0 (f) and GM-38 (g) were treated with 0 (Control) or 100 nM colchicine for 24 h and fixed and probed for β-tubulin (yellow) and nuclei stained with DAPI (blue). Objective (× 100), scale bar, 20 μm, white arrow denotes polynucleation. (h) 786-0s were treated as indand 48 h after infection, nonpermeabilized cells were stained with PI and sorted by flow cytometry. (i) 786-0s were pretreated with colchicine as above (solid line/white squares) or vehicle (dotted line/black circles) and infected with MOI 0.01 (multistep) or MOI 3 (single step) of VSVΔ51 or wtVSV, and supernatants were titred by plaque assay. Fora–c,h–i, error bars or numbers represent s.e. from at least three independent experiments. The compounds, their drug class and structures are listed in Supplementary Table 1 . To validate their activity, we selected representative members of the colchicinoid (colchicine), vinka alkaloid (vinorelbine) and benzimidazole (nocodazole, albendazole and parbendazole) drug classes. These MDAs were tested across a range of concentrations on VSVΔ51-resistant 786-0 human renal carcinoma cells ( Fig. 1a ). Viability assays using alamarBlue metabolic dye revealed that all five drugs enhanced cell killing elicited by a low multiplicity of infection of VSVΔ51 (MOI=0.01, Fig. 1a ). Similar results were obtained in VSVΔ51-resistant mouse cancer cell lines (4T1 and CT26, Supplementary Fig. 1a,b ). Treatment of cancer cells with colchicine, a drug used for autoinflammatory diseases such as gouty arthritis [15] and one of the most potent MDAs tested, led to synergistic killing in combination with both VSVΔ51 and wtVSV ( Supplementary Fig. 1c ). Colchicine also robustly enhanced the activity of Maraba MG-1, an IFN-sensitive onocolytic rhabdovirus strain closely related to VSVΔ51 (ref. 16 ; Supplementary Fig. 1d ). In contrast, MDAs did not enhance VSVΔ51-mediated killing in normal human fibroblasts at any dose tested (GM-38 cells, Fig. 1b ). Figure 1: MDAs enhance VSVΔ51 spread in cancer but not normal cells. ( a , b ) 786-0 cancer ( a ) and GM-38 normal ( b ) cells were pretreated with MDAs ( x axis) and then challenged with VSVΔ51, MOI 0.01. Forty-eight hours later, cell viability was assessed. ( c ) 786-0, U251 and 4T1 cancer cells as well as GM-38 were pretreated with colchicine ( x axis) and infected as above for 48 h and supernatants titred. ( d , e ) 786-0 and GM-38 cells were treated with 100 nM colchicine or vehicle before infection with VSVΔ51-GFP or wtVSV, as above. At 48 h post infection, phase contrast and fluorescent images were taken ( e , scale bar, 50 μm), and cell lysates subject to western blot, where VSV proteins are indicated by arrows ( d ). ( f , g ) 786-0 ( f ) and GM-38 ( g ) were treated with 0 (Control) or 100 nM colchicine for 24 h and fixed and probed for β-tubulin (yellow) and nuclei stained with DAPI (blue). Objective (× 100), scale bar, 20 μm, white arrow denotes polynucleation. ( h ) 786-0s were treated as in d and 48 h after infection, nonpermeabilized cells were stained with PI and sorted by flow cytometry. ( i ) 786-0s were pretreated with colchicine as above (solid line/white squares) or vehicle (dotted line/black circles) and infected with MOI 0.01 (multistep) or MOI 3 (single step) of VSVΔ51 or wtVSV, and supernatants were titred by plaque assay. For a – c , h – i , error bars or numbers represent s.e. from at least three independent experiments. Full size image MDAs and rhabdovirus infection can independently have cytotoxic effects. We considered that the visible synergy between drug and rhabdoviruses could, therefore, result from improved rhabdovirus spread/oncolysis, increased sensitivity to MDAs or both. Microtubule destabilization using colchicine and other MDAs robustly increased VSVΔ51-GFP (green fluorescent protein) spread as well as viral titres in several human and mouse cancer cell lines but not in normal fibroblasts, consistent with a cancer-specific enhancement of viral growth ( Fig. 1c,e and Supplementary Fig. 1e,f ). In cancerous 786-0, but not in normal GM-38 cells, colchicine increased VSVΔ51-GFP spread ( Fig. 1c,e ) and viral protein expression ( Fig. 1d ). Immunofluorescence staining for β-tubulin revealed that colchicine effectively depolymerized microtubules in both cell lines at 100 nM, a dose prominently effective at enhancing rhabdovirus activity in cancer cells ( Fig. 1f,g ). Indeed, the increase in viral spread in 786-0 cells was observed specifically at the doses at which microtubule disruption by colchicine was visible, suggesting that the effects of MDA treatment on virus spread and cytotoxicity are dependent on destabilization of microtubule structures ( Supplementary Figs 2 and 7a ). Furthermore, this correlation was observed whether or not colchicine was left in or removed before VSVΔ51 infection ( Supplementary Fig. 2 ). Colchicine treatment also led to increased numbers of polynucleate, giant cells in 786-0 but not in normal GM-38 ( Fig. 1f versus Fig. 1g (arrow), Supplementary Fig. 2 ). Comparing multi-step and single-step virus growth profiles suggests that in cancer cells, microtubule destabilization has an impact on the ability of VSVΔ51 to spread as opposed to its replication rate ( Fig. 1i ). In contrast, a slightly negative effect of the drug on virus propagation was observed using wtVSV ( Fig. 1d,h,i ). In parallel, we quantified cells positive for virally expressed GFP and propidium iodide (PI) staining using flow cytometry. PI staining was performed without permeabilizing the cells such as to identify dead or dying PI-positive cells. This confirmed that, while wtVSV propagation is hampered by colchicine treatment (fewer GFP-positive cells, Fig. 1h ), cell death is nonetheless increased in comparison with virus or drug alone (more PI-positive cells, Fig. 1h ), consistent with results from synergy assays ( Supplementary Fig. 1c ). The combination of VSVΔ51 and colchicine also led to substantially more PI-positive cells than either treatment alone, although this was accompanied by substantially increased GFP-positive infected cells in sharp contrast with wtVSV ( Fig. 1h ). Altogether, these data suggest that MDAs enhance rhabdovirus-mediated oncolysis through dual effects on viral spread and cell death. In the case of IFN-sensitive mutants such as VSVΔ51, these effects converge potently to kill resistant cancer cells while leaving normal cells unharmed. Microtubule disruption enhances oncolytic rhabdoviruses In order to eliminate the possibility that MDAs can synergize with rhabdoviruses in cancer cells through off-target effects, we obtained A549-T12 (AT12) and -T24 (AT24) cells, which have become resistant to the effects of Taxol through a mutation, rendering them dependent on Taxol in order for their microtubules to remain stable [17] . Indeed, tubulin staining of AT12 grown in the absence of Taxol reveals weak microtubule architecture and evidence of polynucleation compared with AT12 maintained in Taxol-containing media ( Supplementary Fig. 3a ). Similarly to other cancer cell lines, in parental A549 cells we observed that colchicine-induced microtubule disruption could significantly increase VSVΔ51-GFP spread and viral titres ( Supplementary Fig. 3b–d ). Supporting a role for microtubule destabilization, VSVΔ51-GFP spread and viral titres were significantly increased in AT12 and AT24 deprived of Taxol with destabilized microtubules compared with cells grown with Taxol where microtubule architecture was preserved ( Supplementary Fig. 3e,f ). To address this further, we derived three colchicine-resistant 786-0 sublines (786-0 CRV1-3), in the presence of 10 μg ml −1 verapamil to prevent P-glycoprotein-mediated efflux of colchicine [18] . Correlating with visibly reduced cytotoxicity ( Supplementary Fig. 4a , phase contrast), colchicine treatment of 786-0 CRV cells had no effect on viral spread determined by GFP quantification or viral titres ( Supplementary Fig. 4a–c ). Taken together, our data suggest that the enhancing effects of MDAs on oncolytic rhabdovirus activity are strongly linked to microtubule destabilization as opposed to off-target effects. Efficacy of combined MDA and OV treatments in vivo Since colchicine, vinorelbine and other MDAs enhanced oncolytic rhabdovirus efficacy in vitro , we evaluated the potential therapeutic benefit of combined MDA/oncolytic rhabdovirus in vivo in a series of xenograft, syngeneic and transgenic mouse tumour models. Human HT29 colon tumour xenografts were robustly sensitized to intratumorally (i.t.) delivered oncolytic MG-1 (10 8 plaque-forming units or p.f.u.) following intraperitoneal (i.p.) administration of colchicine (2 mg kg −1 ). In this model, combination therapy led to substantially delayed tumour progression compared with either monotherapy ( Fig. 2a ). Similar results were obtained using VSVΔ51 in a syngeneic mouse colon cancer model ( Supplementary Fig. 5d ). In a more highly virus-refractory and aggressive subcutaneous 4T1 syngeneic model of triple-negative breast cancer, co-administration of VSVΔ51 (10 8 p.f.u. i.t.) and vinorelbine (8 mg kg −1 ) or colchicine (2 mg kg −1 ) i.p led to delayed tumour progression and significantly prolonged survival compared with monotherapies alone ( Fig. 2d , Supplementary Fig. 5a ). Similar effects were observed using MG-1 in this model ( Supplementary Fig. 5b ). B16/F10 melanoma tumours implanted orthotopically in syngeneic Bl/6 mice were analogously sensitized to VSVΔ51 oncolytic activity following co-treatment with colchicine. While neither monotherapy had any measurable impact, the combination therapy had a significant effect in prolonging survival in this highly aggressive model ( Supplementary Fig. 5c ). 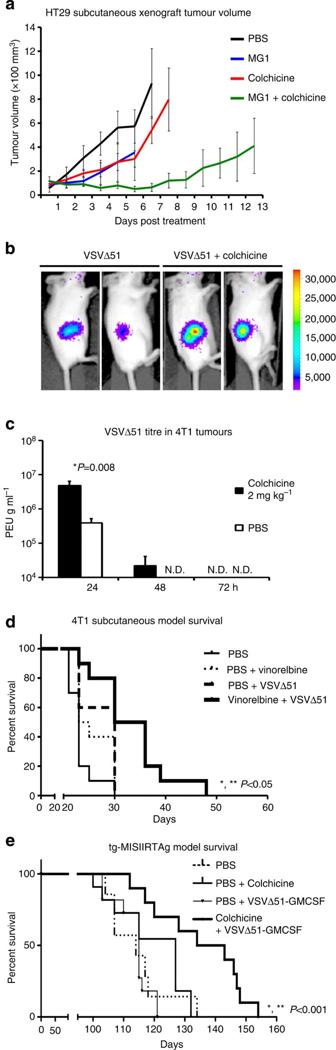Figure 2: Colchicine increases VSVΔ51 spread and oncolytic activity in resistant syngeneic and transgenic tumour models. (a) Human colon carcinoma HT29 cells were established in nude mice. Ten days later, mice were treated with colchicine, MG-1, a combination of MG-1 and colchicine or with PBS only. Tumour volume was monitored for each group and average tumour volumes are shown (N=4–5). Error bars correspond to the s.e. (b) 4T1 tumour-bearing syngeneic mice were treated with VSVΔ51-luciferase or PBS, and colchicine or vehicle and luminescence monitored after 24 h. (c) 4T1 tumours (N=5) from mice treated as inbwere harvested at the indicated times and titred by plaque assay (*P<0.05,t-test; ND=not detected). (d) 4T1 tumour-bearing syngeneic mice were treated with VSVΔ51, vinorelbine, a combination of VSVΔ51 and vinorelbine or PBS (N=10 per group). Survival was monitored over time. Log-rank test indicates that the combined treatment is significantly prolonged over virus alone (*P=0.024) or drug alone (**P=0.0082). (e) tgMISSIIR-TAg transgenic mice were treated with VSVΔ51-GM-CSF (n=11), PBS (n=7) colchicine (n=11) or VSVΔ51-GM-CSF and colchicine (n=10). Survival was monitored over time. Log-rank test indicates that the combined treatment is significantly prolonged over colchicine (*P=0.0082) and VSVΔ51-GM-CSF (**P=0.0007) alone. Figure 2: Colchicine increases VSVΔ51 spread and oncolytic activity in resistant syngeneic and transgenic tumour models. ( a ) Human colon carcinoma HT29 cells were established in nude mice. Ten days later, mice were treated with colchicine, MG-1, a combination of MG-1 and colchicine or with PBS only. Tumour volume was monitored for each group and average tumour volumes are shown ( N =4–5). Error bars correspond to the s.e. ( b ) 4T1 tumour-bearing syngeneic mice were treated with VSVΔ51-luciferase or PBS, and colchicine or vehicle and luminescence monitored after 24 h. ( c ) 4T1 tumours ( N =5) from mice treated as in b were harvested at the indicated times and titred by plaque assay (* P <0.05, t -test; ND=not detected). ( d ) 4T1 tumour-bearing syngeneic mice were treated with VSVΔ51, vinorelbine, a combination of VSVΔ51 and vinorelbine or PBS ( N =10 per group). Survival was monitored over time. Log-rank test indicates that the combined treatment is significantly prolonged over virus alone (* P =0.024) or drug alone (** P =0.0082). ( e ) tgMISSIIR-TAg transgenic mice were treated with VSVΔ51-GM-CSF ( n =11), PBS ( n =7) colchicine ( n =11) or VSVΔ51-GM-CSF and colchicine ( n =10). Survival was monitored over time. Log-rank test indicates that the combined treatment is significantly prolonged over colchicine (* P =0.0082) and VSVΔ51-GM-CSF (** P =0.0007) alone. Full size image As expected from in vitro evidence ( Fig. 1a–i ), the effects of colchicine were associated with tumour-specific increases in OV growth. Using a firefly luciferase-expressing VSVΔ51 and an in vivo imaging system (IVIS), we observed that 24 h post infection (i.t), 4T1-grafted animals treated with colchicine exhibited increased luminescence specifically in tumours ( Fig. 2b ). Consistent with this, a significant increase in VSVΔ51 titres was observed in colchicine-treated animals ( Fig. 2c ). In contrast, assessment of viral titres in normal organs including the spleen, heart, liver, lungs, kidney and brain by standard plaque assay revealed no detectable VSVΔ51 in any organ at any time point in both PBS- and colchicine-treated mice. The efficacy of combined rhabdovirus/MDA treatment was subsequently evaluated in a highly treatment-resistant tgMISIIR-TAg transgenic ovarian cancer mouse model. These mice express SV40 Large T-antigen specifically in the ovaries and develop palpable tumours at 10–11 weeks [19] , [20] . In these experiments, we used VSVΔ51-expressing granulocyte–macrophage colony-stimulating factor (GM-CSF) to further increase antitumour activity. Figure 2e shows that weekly treatment cycles of VSVΔ51-GM-CSF and colchicine both delivered i.p. led to significantly prolonged survival of tgMISIIR-TAg mice as compared with either monotherapy. Overall, these data suggest that combined oncolytic rhabdovirus and MDA treatment can significantly increase antitumour efficacy, prolonging survival even in highly treatment-resistant spontaneously arising tumours. MDAs alter the type I IFN response Combined treatment with MDAs and VSVΔ51 enhanced viral spread and oncolysis, providing therapeutic benefit in several resistant murine cancer models. We therefore used gene expression microarrays to gain insight into the possible mechanisms involved. We looked at gene expression profiles of 786-0 cells 24 h following VSVΔ51 or mock infection in presence and absence of 100 nM colchicine. In our analysis, we identified a subset of 248 genes that was either up- or down -regulated (more than twofold, P <0.05) in VSVΔ51-infected cells exclusively in the absence of drug ( Fig. 3a ). On the basis of gene set-enrichment analyses using both GOrilla and DAVID gene set databases [21] , [22] , [23] , [24] , this group of 248 genes, and more specifically the 158 virus-induced genes dampened by colchicine, is significantly enriched in type I IFN-responsive genes ( Fig. 3a , lower inset and Fig. 3b ). 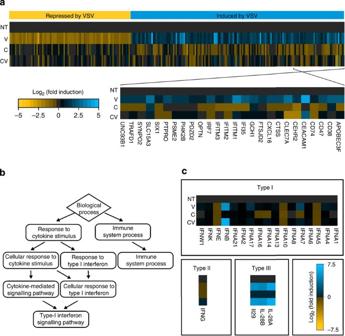Figure 3: Microtubule destabilization hinders the response to type I IFN-stimulated genes induced by VSVΔ51. (a) 786-0 cells were pretreated with 100 nM colchicine or vehicle and infected with VSVΔ51 at MOI 0.01 or were mock-infected. Twenty-four hours later, RNA was collected and pooled, and triplicate experiments were hybridized on Affymetrix human Gene ST 1.0 microarrays. Shown are heat maps of all genes found to be significantly increased (blue) or decreased (yellow) more than twofold in VSVΔ51-infected 786-0 as compared with control (NT), VSV-infected (V), colchicine-treated (C) and colchicine-treated, virus-infected (V+C) conditions (P<0.05,Z-test). Inset shows a group of type I IFN-stimulated genes that are upregulated in V but not V+C conditions. (b) Summary of gene ontology relationships for enriched gene sets froma. (c) Microarray expression data for a subset of interferon isoforms and subtypes froma. Figure 3: Microtubule destabilization hinders the response to type I IFN-stimulated genes induced by VSVΔ51. ( a ) 786-0 cells were pretreated with 100 nM colchicine or vehicle and infected with VSVΔ51 at MOI 0.01 or were mock-infected. Twenty-four hours later, RNA was collected and pooled, and triplicate experiments were hybridized on Affymetrix human Gene ST 1.0 microarrays. Shown are heat maps of all genes found to be significantly increased (blue) or decreased (yellow) more than twofold in VSVΔ51-infected 786-0 as compared with control (NT), VSV-infected (V), colchicine-treated (C) and colchicine-treated, virus-infected (V+C) conditions ( P <0.05, Z -test). Inset shows a group of type I IFN-stimulated genes that are upregulated in V but not V+C conditions. ( b ) Summary of gene ontology relationships for enriched gene sets from a . ( c ) Microarray expression data for a subset of interferon isoforms and subtypes from a . Full size image At first glance, our data suggested that microtubule destabilization has an impact on the transcriptional response to type I IFN normally induced following infection. However, the type I IFN response is thought to proceed in three waves. First, activation of pattern recognition receptors such as Toll-like receptor 3 and Retinoic acid-induced gene I, through signalling via Tank-binding kinase 1/IκB kinase ε (TBK-1/IKKε) and transcription factor IFN regulatory factor 3 (IRF-3) leads to increased ‘first-wave’ IFNβ transcription, translation, and secretion. Second, autocrine and paracrine signalling through type I IFN receptor (IFNR)/Janus kinase (JAK)/STAT (Signal Transducer and Activator of Transcription) leads to the formation of Interferon Stimulated Gene Factor 3, and to the upregulation of IFN-stimulated genes (ISGs) including IRF-7 and ‘second-wave’ IFNα isoforms. Third, additional ISGs are upregulated because of the combination of persistent IFN signalling and IRF-7 upregulation [7] , [25] . Closer inspection of the microarray data revealed that, while the induction of second-wave IFNα isoforms was dampened after treatment with colchicine, the induction of first-wave IFNβ mRNA remained similar ( Fig. 3c ). This was confirmed by looking at IFNβ mRNA expression in both nuclear and cytoplasmic compartments by real-time PCR ( Fig. 4a ). This suggested that virus-induced signalling leading to IFNβ mRNA upregulation as well as its subsequent cytoplasmic export is not affected by the MDA treatment. Further supporting this, IRF-3 nuclear shuttling and its phosphorylation status was unchanged by the colchicine treatment shortly following VSVΔ51 infection at high MOI ( Fig. 4b ). 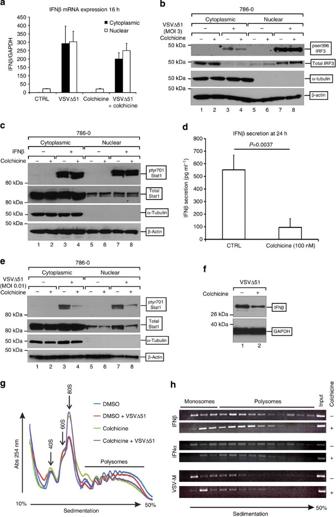Figure 4: Microtubule destabilization leads to a decrease in type I IFN production. (a) 786-0 cells were pretreated with 100 nM colchicine or vehicle and infected with VSVΔ51 at MOI 0.01 or mock. Sixteen hours later, qPCR was performed with cDNA from nuclear and cytoplasmic fractions. Data represent the fold change in IFN-β, normalized to GAPDH, relative to uninfected controls. (b) 786-0 were treated as above and infected at MOI 3 or mock. Eight hours later, fractionated lysates were probed with the indicated antibodies. (c) 786-0 cells were pretreated with colchicine and challenged with 0 or 500 U ml−1IFNβ. One hour later, fractionated cell lysates were probed with the indicated antibodies. 786-0 cells were treated as inaand 24 h later (d) supernatants were collected and IFN-β quantified by ELISA, (e,f) 786-0 pretreated as inaand cell lysates probed for the indicated antibodies. (g,h) 786-0 cells were treated as inaand at 24 h post infection, whole-cell lysates were collected and run on a 10–50% sedimentation gradient and absorbance measured over each fraction. (h) cDNA was generated from fractions and the abundance of mRNAs encoding IFNα, IFNβ and VSV M in each fraction assessed with PCR. Fora,d, error bars represent s.e. from at least three replicate experiments and data analysed by analysis of variance (ANOVA) for statistical significance (P<0.05). Forb,c,e,f, representative blots from three experiments are shown and apparent molecular sizes (kDa) of the prestained protein ladder (26616, Thermo Scientific) according to electrophoresis conditions are marked on the left. Figure 4: Microtubule destabilization leads to a decrease in type I IFN production. ( a ) 786-0 cells were pretreated with 100 nM colchicine or vehicle and infected with VSVΔ51 at MOI 0.01 or mock. Sixteen hours later, qPCR was performed with cDNA from nuclear and cytoplasmic fractions. Data represent the fold change in IFN-β, normalized to GAPDH, relative to uninfected controls. ( b ) 786-0 were treated as above and infected at MOI 3 or mock. Eight hours later, fractionated lysates were probed with the indicated antibodies. ( c ) 786-0 cells were pretreated with colchicine and challenged with 0 or 500 U ml −1 IFNβ. One hour later, fractionated cell lysates were probed with the indicated antibodies. 786-0 cells were treated as in a and 24 h later ( d ) supernatants were collected and IFN-β quantified by ELISA, ( e , f ) 786-0 pretreated as in a and cell lysates probed for the indicated antibodies. ( g , h ) 786-0 cells were treated as in a and at 24 h post infection, whole-cell lysates were collected and run on a 10–50% sedimentation gradient and absorbance measured over each fraction. ( h ) cDNA was generated from fractions and the abundance of mRNAs encoding IFNα, IFNβ and VSV M in each fraction assessed with PCR. For a , d , error bars represent s.e. from at least three replicate experiments and data analysed by analysis of variance (ANOVA) for statistical significance ( P <0.05). For b , c , e , f , representative blots from three experiments are shown and apparent molecular sizes (kDa) of the prestained protein ladder (26616, Thermo Scientific) according to electrophoresis conditions are marked on the left. Full size image We next looked for potential effects of MDAs on signalling downstream of IFNβ secretion. Colchicine treatment at 100 nM did not inhibit STAT-1 phosphorylation or alter nuclear/cytoplasmic distribution of the transcription factor following treatment with exogenous IFNβ ( Fig. 4c ), indicating fully functional IFN response through the (IFNR)/JAK/STAT pathway. Consistent with this, colchicine treatment (100 nM) could not overcome the antiviral effects of type I IFNs in either 786-0 or U251 cells ( Supplementary Fig. 6a,b ), in sharp contrast with suberoyl anilide hyroxamic acid, an HDAC inhibitor known to effectively dampen the antiviral effects of type I IFNs ( Supplementary Fig. 6a and ref. 13 ). Overall, this suggests that MDAs severely dampen the type I IFN response without affecting signalling upstream of IFNβ mRNA induction or modulating signalling downstream of the antiviral cytokine. MDAs inhibit translation of type I IFN mRNA Altogether, our data suggested that microtubule destabilization decouples first- and second-wave antiviral responses without altering the intracellular signalling pathways known to be involved in their induction. We considered that this phenomenon could be explained if MDAs have an impact on type I IFN secretion, and in particular that of first-wave IFNβ. We addressed this possibility directly using enzyme-linked immunosorbent assay (ELISA). Even though mRNA levels and subcellular distribution were unaltered ( Figs 3c and 4a ), treatment with 100 nM colchicine caused a significant decrease in secreted IFNβ following a 24-h infection with a low MOI of VSVΔ51 ( Fig. 4d ). Furthermore, exposure of 786-0 to increasing doses of colchicine uncovered a correlation between microtubule disruption ( Supplementary Fig. 2 ), inhibition of IFNβ secretion and increased virus titres ( Supplementary Fig. 7a ). A similar effect on IFNβ secretion was observed using other MDAs ( Supplementary Fig. 8c ). In contrast, VSVΔ51-induced IFNβ secretion in colchicine-resistant, 786-0 colchicine resistant variant (CRV) sublines, was not hampered by colchicine ( Supplementary Fig. 7b ). A time course revealed that microtubule destabilization effectively delayed the onset of IFNβ production, which eventually accumulated over 48 h in infected cell culture supernatants ( Supplementary Fig. 8a ). Consistent with microarray mRNA expression data ( Fig. 3c ), IFNα was detected at lower concentrations than IFNβ following infection, and treatment with colchicine further reduced this ( Supplementary Fig. 8b ). In line with the observed decrease in type I IFN secretion, we found that the colchicine treatment reduced phosphorylation of STAT-1 24 h post infection ( Fig. 4e ). As was observed in 786-0 cells, IFNβ secretion was also inhibited by colchicine in U251 cancer cells ( Supplementary Fig. 8d ). However, the colchicine treatment also decreased IFNβ secretion in normal MRC-5 fetal lung fibroblasts ( Supplementary Fig. 8d ), suggesting that this effect is not restricted to cancer cells and that additional mechanisms may contribute to the cancer-specific enhancement in VSVΔ51 spread observed in vitro and in vivo . Given that microtubules are known to play a role in vesicular transport and that microtubule destabilizers such as colchicine have been shown to have an impact on the secretion of various proteins [26] , [27] , [28] , [29] , [30] , we considered the possibility that microtubule destabilization may simply have an impact on the ability of cells to secrete cytokines in response to virus infection. To assess this, we looked at the impact of microtubule destabilization on overall protein secretion using 35 S pulse-labelling following challenge with either VSVΔ51, G-less VSVΔ51 (which can infect but cannot exit the cell) or treatment with the Toll-like receptor agonist poly (I:C). Visualizing protein secretion patterns by autoradiogram, we observed a variety of responses to the colchicine treatment following viral stimulation. Whereas the secretion of some proteins 24 h post infection was increased by all three stimuli but reduced following treatment with colchicine (analogously to what was observed by ELISA for IFNβ and α), other proteins were not influenced by any viral stimulus nor affected by colchicine ( Supplementary Fig. 8e ). This argues against a systematic negative impact of microtubule destabilization on protein secretion. To further address this, we quantified interleukin (IL)-6 secretion in cell supernatants 24 h following VSVΔ51 infection in presence and absence of colchicine, given that similarly to IFNβ this cytokine was robustly upregulated by VSVΔ51 infection at the mRNA level on the basis of microarray analyses ( Fig. 3c and Supplementary Table 2 ). In sharp contrast with what was observed for type I IFNs, these experiments revealed no significant decrease in virus-induced IL-6 secretion following treatment with colchicine ( Supplementary Fig. 8f ). Further arguing against systematic inhibition of protein secretion following microtubule destabilization, secreted mouse GM-CSF encoded by the VSVΔ51-GM-CSF virus used for in vivo experiments shown in Fig. 2e increased proportionally to viral titres upon treatment with colchicine ( Supplementary Fig. 8g ). We considered the possibility that microtubule disruption leads to decreased secretion of type I IFNs indirectly by reducing the translation of their mRNAs. Supporting this idea, western blots on whole-cell extracts of infected 786-0 cells revealed that at 24 h post infection, intracellular IFNβ protein expression levels decrease in parallel with the observed reduction in protein secretion ( Fig. 4f , Supplementary Fig. 8a,d ). To measure translation efficiency, we looked at RNA distribution in monoribosomes and polyribosomes using gradient sedimentation. Figure 4g shows that the colchicine treatment of 786-0 cells, irrespective of infection, led to a shift in mRNA distribution from polysome (highly translated) to monosome (poorly translated) fractions, albeit to a lesser extent than PP242, an mammalian target of rapamycin (mTOR) and translation inhibitor (see Supplementary Fig. 9a ). Assessment of mRNA abundance by semiquantitative PCR further showed that both IFNβ and IFNα were less abundant in the highest-density polysomes of colchicine-treated cells ( Fig. 4h ). In contrast, looking at VSV M revealed a slight increase in lower-density polysomes upon treatment with colchicine ( Fig. 4h ). However, we failed to observe any alterations in the expression or phosphorylation of either mTOR target 4E-BP1 or downstream S6K target rpS6 (ref. 31 ) following treatment of 786-0 cells with colchicine ( Supplementary Fig. 9a,b ) arguing against a role of mTOR or 4E-BP in mediating the observed effects of MDAs on type I IFN mRNA translation efficiency. Overall, this suggests that microtubule destabilization reduces translation efficiency of cellular mRNAs such as type I IFNs, while permitting translation of viral genes. MDAs enhance bystander death by virus-induced cytokines While the data thus far shed light on the mechanisms leading to the enhancement of VSVΔ51 spread in cancer cells, it remained unclear why MDAs could also increase rhabdovirus infection-associated cell death ( Fig. 1a,h ). We therefore assessed whether viral triggers could be sufficient to elicit cytotoxic effects upon microtubule destabilization. To this end, we challenged colchicine or vehicle-treated 786-0 cells with a UV-inactivated wtVSV. As expected, even at a very high MOI (200) UV-inactivated wtVSV did not affect viability of 786-0 cells in control conditions. However, UV-inactivated virus was capable of effectively killing 786-0 cells treated with colchicine (starting at MOI 50, Fig. 5a ). This was also observed in mouse 4T1 cells, albeit starting at a higher MOI of UV-inactivated virus ( Supplementary Fig. 10a ). 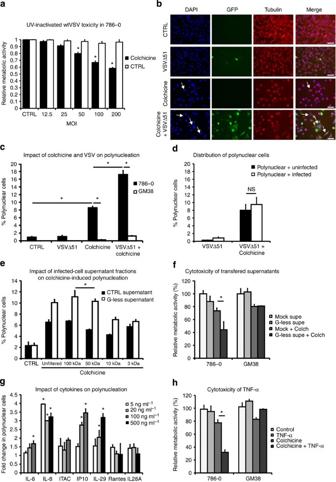Figure 5: VSV-induced cell death is increased by secreted factors that lead to polynucleation and death, specifically in cancer cells. (a) 786-0 were treated with 100 nM colchicine or vehicle and challenged with UV-inactivated virus (xaxis). Cell viability was assessed after 48 h. (b–d) 786-0 and GM-38 were pretreated with colchicine as above and infected with VSVΔ51-GFP, MOI 0.01 or were mock-infected. After 24 h, cells were fixed and stained with DAPI and anti-β-tubulin (red). Fluorescence microscopy pictures were taken at × 40 (b, scale bar, 50 μm) and GFP-positive and polynuclear cells scored (yellow arrows andc). (d) 786-0 polynucleation data fromcanalysing virus-infected (GFP-positive) and uninfected cells. (e) 786-0 cells were infected with G-less VSVΔ51-GFP at MOI 10, and 24 h later supernatants were passed through cutoff filters (xaxis) and applied directly to virus-naive 786-0 cells treated with colchicine or vehicle. Twenty-four hours later, cells were fixed and stained with DAPI, and β-tubulin and polynuclear cells counted. (f) 786-0 and GM-38 cells were treated as ineand cell viability was assessed. (g) 786-0 cells were pretreated with colchicine and recombinant cytokines (xaxis). Twenty-four hours later, polynuclear cells were counted. (h) 786-0 or GM-38 treated with TNFα with colchicine or vehicle and cell viability assessed. Error bars represent s.e. from at least three replicate experiments and data analysed by ANOVA for statistical significance (*P<0.05). Figure 5: VSV-induced cell death is increased by secreted factors that lead to polynucleation and death, specifically in cancer cells. ( a ) 786-0 were treated with 100 nM colchicine or vehicle and challenged with UV-inactivated virus ( x axis). Cell viability was assessed after 48 h. ( b – d ) 786-0 and GM-38 were pretreated with colchicine as above and infected with VSVΔ51-GFP, MOI 0.01 or were mock-infected. After 24 h, cells were fixed and stained with DAPI and anti-β-tubulin (red). Fluorescence microscopy pictures were taken at × 40 ( b , scale bar, 50 μm) and GFP-positive and polynuclear cells scored (yellow arrows and c ). ( d ) 786-0 polynucleation data from c analysing virus-infected (GFP-positive) and uninfected cells. ( e ) 786-0 cells were infected with G-less VSVΔ51-GFP at MOI 10, and 24 h later supernatants were passed through cutoff filters ( x axis) and applied directly to virus-naive 786-0 cells treated with colchicine or vehicle. Twenty-four hours later, cells were fixed and stained with DAPI, and β-tubulin and polynuclear cells counted. ( f ) 786-0 and GM-38 cells were treated as in e and cell viability was assessed. ( g ) 786-0 cells were pretreated with colchicine and recombinant cytokines ( x axis). Twenty-four hours later, polynuclear cells were counted. ( h ) 786-0 or GM-38 treated with TNFα with colchicine or vehicle and cell viability assessed. Error bars represent s.e. from at least three replicate experiments and data analysed by ANOVA for statistical significance (* P <0.05). Full size image MDAs are well known to induce mitotic catastrophe and polynucleation, killing cells that divide rapidly and that have lost cell cycle checkpoints, two key hallmarks of cancer [32] . To gain a better understanding of the mechanisms leading to increased death in MDA-treated cells challenged with rhabdovirus, we looked at the frequency of polynuclear cells in the context of infection. We treated 786-0 cells with 100 nM colchicine or vehicle and infected them with VSVΔ51-GFP at low MOI (0.01). Twenty-four hours post infection, cells were fixed and stained with a nuclear dye (4',6-diamidino-2-phenylindole, DAPI) and an anti-β-tubulin antibody. Fluorescence microscopy was then used to visualize and count GFP-positive infected cells and those exhibiting characteristic polynucleation (see Fig. 1f white arrow and Supplementary Fig. 10b ). As expected, the colchicine treatment led to increased polynuclear cells, whereas infection with VSVΔ51-GFP alone did not. Importantly, upon co-treatment with VSVΔ51-GFP and colchicine, 786-0 cells exhibited a robust increase in the number of virus-associated GFP-positive cells and a near doubling in the number of polynucleated cells compared with cells treated with colchicine alone ( Fig. 5b,c ). Dose–response experiments revealed that this effect is observed starting at doses corresponding to those at which microtubule destabilization, decreased IFNβ secretion, and increased virus spread are also observed ( Supplementary Figs 2a,b, 7a and 10c ). In contrast, polynucleation remained low in normal GM-38 cells under these conditions ( Fig. 5c ). Moreover, looking at the proportion of polynuclear 786-0 cells in infected (GFP+) and uninfected (GFP−) populations following the colchicine treatment further revealed that these were equally frequent in infected and uninfected cells ( Fig. 5d ). This distribution suggested the likely involvement of a virus-induced secreted factor in promoting polynucleation in the entire colchicine-treated 786-0 cell population. To explore this idea, we used supernatants from 786-0 cells infected with G-less VSVΔ51-GFP. As described previously, G-less VSVΔ51-GFP can infect and replicate but cannot bud from the cytoplasmic membrane [33] . We infected 786-0 cells with G-less VSVΔ51-GFP at high MOI (10) or naught and collected supernatants 24 h post infection. These supernatants were applied to virus-naive 786-0 cells treated with 100 nM colchicine or vehicle, and 24 h later cellular polynucleation was quantified. Consistent with the involvement of a secreted factor, supernatants from G-less VSVΔ51-infected but not mock-treated cells increased polynucleation and cell death in virus-naive 786-0 cells treated with colchicine ( Fig. 5e,f ). However, this did not occur when the same experiments were repeated using normal GM-38 supernatants and cells ( Fig. 5f ). Pointing to the involvement of one or more secreted factors between 10 and 50 kDa ( Fig. 5e ), the polynucleation-inducing activity of G-less VSVΔ51-infected 786-0 cell supernatants was abrogated following filtration using a 10-kDa- but not 50- or 100-kDa molecular-weight cutoff filter. To generate a list of candidates, we queried the microarray data looking for secreted proteins between 10 and 50 kDa induced by VSVΔ51 in both vehicle- and colchicine-treated conditions. The short list of these candidates is shown in Supplementary Table 2 . In addition to type I IFNs, this included several growth-promoting cytokines (for example, Rantes, IP-10, CXCL11, IL-8 and IL-6) as well as death-inducing cytokines (for example, tumour necrosis factor (TNF)-α and other TNF-related proteins). Type III IFNs (IL-28a, IL-28b and IL-29) also figured on this list. While it is likely that many of these factors work in concert to recapitulate the synergy observed between virus infection and colchicine treatment observed in Fig. 5a–f , we nevertheless evaluated the impact of a subset of cytokines on the frequency of polynuclear cells in 786-0 cells in presence of colchicine. We found that some cytokines such as IL-6, IL-8, IP-10 and IL-29 significantly increased the frequency of polynuclear cells in colchicine-treated 786-0 cells ( Fig. 5g ). In addition, colchicine treatment increased cell death induced by TNF-α in 786-0 but not GM-38 cells ( Fig. 5h ). Overall, this suggests that infection with rhabdoviruses in the presence of colchicine leads to cancer-specific increases in bystander polynucleation and cell death, likely through the combined action of multiple secreted factors and death-inducing cytokines. In this study, we reveal that MDAs can act synergistically with oncolytic rhabdoviruses by decreasing antiviral type I IFN production and increasing virus-induced cytokine-mediated bystander killing (see diagram summary in Fig. 6a,b ). While we show here that MDAs elicit these two effects simultaneously, further dissecting their individual influences can provide deeper understanding on their interplay and contribution to the observed phenomena. Our data suggest that both effects are intimately linked to microtubule destabilization (see Supplementary Figs 2a,b, 7a and 10c ), making this difficult to address this experimentally. To get around this problem, we adapted a mathematical model recently developed to investigate the impact of IFN dynamics on oncolytic rhabdovirus activity [11] . The initial framework, which we have previously shown to closely fit experimental data in normal and cancer cells [11] , was modified to model separately or in combination the two effects of MDAs ( Fig. 6c,d and Supplementary Fig. 11a ). 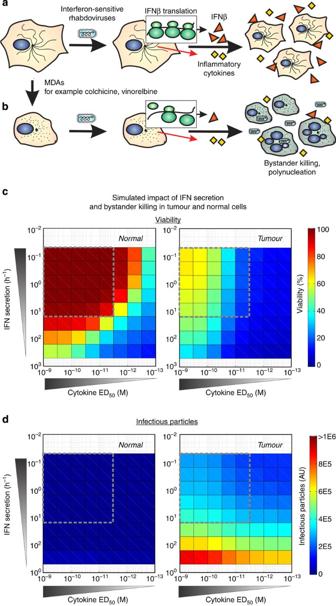Figure 6: Graphical and mathematical models summarizing the synergistic effects of MDAs on oncolytic virotherapy. (a,b) Graphical model. (a) In a subset of cancer cells that are innately resistant to oncolytic rhabdoviruses (for example, VSVΔ51 or MG-1), infection stimulates the production of type I IFN, which hampers viral replication to generate a protected population of cells. (b) Upon treatment with MDAs such as colchicine or vinorelbine, microtubules become destabilized, influencing the translation of cytokines such as IFNβ, by shifting its mRNA distribution from polysome to monosome fractions. This resulting lag in IFNβ secretion boosts viral spread and oncolysis. In addition, MDAs can increase bystander killing attributed to the production of virus-induced inflammatory and cytotoxic cytokines (for example, TNF-α, IL-6, IL-8, IP-10 and IL-29) through a significant increase in the proportion of polynuclear cells, a precedent to mitotic catastrophy and tumour cell destruction. (c,d) Monte Carlo simulations modelling type I IFN secretion decrease, and increased bystander effect, recapitulates the cancer-selective impact of MDAs on VSVΔ51 oncolysis. (c) Heat map summarizing the median viability 72 h post infection in normal or tumour cells as a function of decreasing the rate of IFN release (in a downward direction) and decreasing the ED50 of cytotoxic cytokines (in a rightward direction) in the presence of MDA. (d) Heat map summarizing the median number of free virus particles in the environment 72 h post infection in normal or tumour cells. Figure 6: Graphical and mathematical models summarizing the synergistic effects of MDAs on oncolytic virotherapy. ( a , b ) Graphical model. ( a ) In a subset of cancer cells that are innately resistant to oncolytic rhabdoviruses (for example, VSVΔ51 or MG-1), infection stimulates the production of type I IFN, which hampers viral replication to generate a protected population of cells. ( b ) Upon treatment with MDAs such as colchicine or vinorelbine, microtubules become destabilized, influencing the translation of cytokines such as IFNβ, by shifting its mRNA distribution from polysome to monosome fractions. This resulting lag in IFNβ secretion boosts viral spread and oncolysis. In addition, MDAs can increase bystander killing attributed to the production of virus-induced inflammatory and cytotoxic cytokines (for example, TNF-α, IL-6, IL-8, IP-10 and IL-29) through a significant increase in the proportion of polynuclear cells, a precedent to mitotic catastrophy and tumour cell destruction. ( c , d ) Monte Carlo simulations modelling type I IFN secretion decrease, and increased bystander effect, recapitulates the cancer-selective impact of MDAs on VSVΔ51 oncolysis. ( c ) Heat map summarizing the median viability 72 h post infection in normal or tumour cells as a function of decreasing the rate of IFN release (in a downward direction) and decreasing the ED50 of cytotoxic cytokines (in a rightward direction) in the presence of MDA. ( d ) Heat map summarizing the median number of free virus particles in the environment 72 h post infection in normal or tumour cells. Full size image In agreement with our experimental data with MDAs, this framework predicts that simultaneously decreasing IFN secretion and increasing bystander killing leads to increased viral growth and robust killing of cancer cells, but leaves normal cells unharmed (within a wide range of simulation parameters; Fig. 6c,d , Supplementary Fig. 11b ). However, while decreasing IFN production boosts viral growth preferentially in cancer cells to a certain extent, simulations indicate that increasing bystander killing may be a dominant contributor to the overall cancer-selective cytopathic response when both effects are combined ( Fig. 6c,d , Supplementary Fig. 11b ). Nevertheless, caution must be taken in over-interpreting the results from the model, given the estimates for some of the parameters used may not adequately reflect the underlying biology. Unlike IFN-sensitive VSVΔ51 for which both spread and bystander killing are enhanced by MDAs, wtVSV effectively overcomes the IFN response on its own [6] . This suggests that wtVSV should be mostly prone to the bystander effect of MDAs. It emerges from simulations using our model that increasing bystander killing alone comes at the cost of reducing viral output ( Fig. 6c,d ), corroborating our experimental observations with wtVSV ( Fig. 1h ). Our results altogether suggest that even though VSV has been reported to interact with microtubules in other studies [34] , these cytoskeletal structures are not strictly required for rhabdovirus growth. Rather, our studies and simulations present enhanced bystander killing as an alternative explanation for the moderate inhibition of wtVSV growth measured following treatment of cells with MDAs (Fig. 1i and ref. 34 ). Many viruses, such as vaccinia, are known to exploit the host cytoskeletal system to travel within the cytoplasm and to infect other cells [35] . Suggesting that MDAs may have virus-specific effects, we and others have observed that, while they enhance rhabdoviruses, microtubule destabilizers robustly inhibit vaccinia growth [36] . However, other viruses have been reported to grow at least equivalently in cells with destabilized microtubules. For example, while the mechanism was not addressed, low-dose vinblastine increased the oncolytic activity of herpes simplex virus without affecting viral titres in vitro [37] . It is likely that other IFN-inducing viruses could be enhanced by MDAs by taking advantage of delayed type I IFN secretion. However, our data suggest that rapidly growing viruses such as VSVΔ51 and MG-1 are more likely to benefit given this advantage is only transient (see Supplementary Fig. 8a,b ). Ultimately, this may offer additional selectivity to the approach, reducing the possibility of opportunistic infections that could ensue from hindering the type I IFN system. Somewhat controversial reports dating before the purification and sequencing of type I IFNs in the late seventies [38] noted the impact of drugs such as colchicine and vinblastine on the expression and secretion of antiviral cytokines and several other proteins [26] , [27] , [28] , [29] , [30] . Here we show for the first time direct evidence that several MDAs inhibit type I IFN secretion and provide data supporting the involvement of microtubule destabilization and mRNA translation in this phenomenon. Our results suggest that the incorporation of type I IFN mRNAs in polyribosome structures is compromised following disruption of microtubules. However, only a subset of secreted proteins responded analogously to type I IFNs following the MDA treatment as determined by pulse-chase experiments and by ELISA ( Supplementary Fig. 8e–g ). This brings forth the interesting possibility that microtubules and/or associated factors coordinate efficient translation of a subset of proteins. Supporting this idea, it has been previously reported that microtubule disruption reduces fibronectin mRNA prevalence in polyribosomes of smooth muscle cells [39] . Given these observations, it is tempting to speculate that microtubules coordinate the organization of polyribosome structures, which may be preferentially associated with a subset of mRNAs. Overall, our study shows that MDAs can provide a significant therapeutic benefit when combined with oncolytic rhabdoviruses such as VSVΔ51 and Maraba MG-1, in several models of mouse and human cancers, from various tissue origins, including ovarian, colon, breast and skin (see Fig. 2 and Supplementary Fig. 5 ). While MDAs have been used for decades to treat a number of human ailments including autoimmune disorders, helminthes and cancer [15] , [32] , [40] , one common characteristic is the narrow therapeutic window associated with these agents. In the case of cancer, this has led to the development of more selective biological therapies including therapeutic antibodies and OVs. Therefore, one downside of using classical MDAs in this context is their associated systemic toxicity. Notably, as a strategy to avoid overt toxicity of MDAs, these have been linked to monoclonal antibodies such as Herceptin, which retarget effects towards cancer cells [41] . It will be interesting to test oncolytic rhabdoviruses in combination with novel and recently approved antibody–MDA conjugates for the treatment of cancer in order to take full advantage of the vastly superior selectivity of these therapeutics. Cell lines and culture conditions 4T1 (breast), CT26 (colon), CT26-LacZ (colon) and B16 (melanoma) mouse cancer cells; 786-0 (renal); U251 (glioma), HT29 (colon) human cancer cells; Vero monkey kidney cells; MRC-5 and GM-38 normal human fibroblasts were obtained from the American Type Culture Collection (Manassas, VA). Cells were cultured in HyQ high-glucose Dulbecco’s modified Eagle’s medium (Hyclone, Waltham, MA) supplemented with 10 or 20% (GM-38) fetal calf serum (CanSera, Etobicoke, Ontario, Canada). A549-AT12, A549-AT24 and parental A549 lung carcinoma cells were a kind gift of Dr Susan Horwitz; cells were maintained in RPMI with 10% FBS supplemented with 12 or 24 nM paclitaxel (Taxol; Bristol-Myers Squibb, Princeton, NJ) for AT12 and AT24, respectively. 786-0 CRV were derived through passaging 786-0 cells with 0–10 nM colchicine in the presence of 10 μg ml −1 verapamil (Sigma-Aldrich, St Louis, MO; three or more passages). All cell lines were incubated at 37 °C in a 5% CO 2 -humidified incubator. Viruses, purification and quantification The Indiana serotype of VSV (VSVΔ51 or wild type) was used throughout this study and was propagated in Vero cells. VSVΔ51-expressing GFP, firefly luciferase or murine GM-CSF are recombinant derivatives of VSVΔ51 described previously [7] , [42] . Maraba MG-1 as described in ref. 16 was obtained from Dr David Stojdl. All viruses were propagated on Vero cells and purified on 5–50% Optiprep (Sigma) gradient and all virus titres were quantified by the standard plaque assay on Vero cells as described in ref. 43 . For experiments described in Fig. 5a and Supplementary Fig. 6a , wtVSV was first inactivated by UV crosslinking with a total of 360 mJ cm −2 . Drugs and cytokines Colchicine, vinorelbine, nocodazole, albendazole and parbendazole were obtained from Sigma-Aldrich (St Louis, MO) and dissolved in DMSO. IFNα (Intron A) was obtained from Schering-Plough (Kenilworth, NJ). IFN-β was obtained from PBL Interferon Source (Piscataway, NJ). IL-6, IL-8, ITAC, IP-10, IL-29, IL-28a and TNF-α were obtained from ProSpec Bio (East Brunswick, NJ). In vitro treatment of cells with MDAs and rhabdoviruses Confluent monolayers of cells were pretreated for 2–4 h with drugs, followed by infection with rhabdoviruses at indicated MOIs for the indicated times. Fluorescent images to detect virus replication were obtained using the Axiovert S100 Fluorescence microscope (Carl Zeiss Ltd, Toronto, ON). Cell viability was assessed using an alamarBlue assay (AbD Serotec) according to the manufacturer’s instructions by measuring fluorescence (530 nm excitation and 590 nm emission) on a Fluoroskan Ascent Microplate Fluorometer (Thermo Scientific, Hudson, NH). GFP-fluorescence units were obtained using a Cellomics Arrayscan VTI HCS Reader. Virus titres were determined from cell supernatants by standard plaque assay on Vero cells [43] . Briefly, supernatants were serially diluted and incubated on confluent Vero cells for 45 min. Supernatants were removed and a 1% agarose overlay in Dulbecco’s modified Eagle’s medium (Gibco/BRL) with 20% FBS was immediately added. After 24-h incubation at 37 °C in a 5% CO 2 -humidified incubator, cells were fixed in methanol and stained with a coomassie brilliant blue R (Sigma) solution containing 0.5 g coomassie blue, 20% methanol and 10% acetic acid. Plaques were counted and titres calculated on the basis of the dilution and reported as p.f.u. per ml. Flow cytometry 786-0 cells were plated in 12-well dishes, pretreated with DMSO or 100 nM colchicine for 4 h, followed by mock infection or infection with VSVΔ51-GFP or wtVSV-GFP at MOI 0.01. Forty-eight hours later, cells were collected, washed and resuspended in HBSS containing 10% FBS and 0.01% sodium azide. Nonpermeabilized, single-cell suspensions were labelled with or without 50 μg ml −1 propidium iodide (Sigma) and subjected to flow cytometry on a Beckman Coulter FC500 (data analysed with the Kaluza v1.1 software). Rodent tumour models CT26 and 4T1 models . Six-week-old female Balb/c mice obtained from Charles River Laboratories (Wilmington, MA) were given subcutaneous tumours by injecting ~3 × 10 5 syngeneic 4T1 (or CT26-LacZ) cells suspended in 100 μl PBS. At the indicated times post implantation, tumours were injected with 1 × 10 8 p.f.u. (in 50 μl PBS) of the indicated virus. Four hours later, colchicine or vinorelbine was administered i.p. at the indicated dose. This was repeated a week later for a total of two treatment cycles. Tumour sizes were measured every other day using an electronic caliper. Tumour volume was calculated as=(length × width 2 )/2. For survival studies, mice were culled when tumours had reached 1,600 mm 3 . For in vivo imaging, an IVIS (Perkin Elmer, Waltham, MA) was used as described previously [44] . Briefly, 100 μl of a 10-mg ml −1 D -Luciferin solution in PBS was injected into mice i.p. Five minutes later, mice were anaesthetized using 3% isoflurane and imaged according to the manufacturer’s instructions. For viral quantification described in Fig. 2b , tumours were dissected at the indicated times and homogenized in PBS using a tissue homogenizer before quantification by the standard plaque assay as described above and in ref. 43 . HT29 model . Six-week-old female Nude mice obtained from Charles River Laboratories were injected s.c. with HT29 human colon carcinoma cells (1 × 10 6 ). Ten days later, when tumours reached 5 × 5 mm size, mice were treated with MG-1 i.t. (1 × 10 8 p.f.u.) and/or colchicine i.p. (2 mg kg −1 ). Tumour sizes were measured every other day using an electronic caliper. B16 model . Six-week-old female C57Bl/6 mice obtained from Charles River Laboratories were injected s.c. with B16 melanoma cells (2 × 10 5 ). Two weeks later, when tumours reached 5 × 5 mm size, mice were treated with VSVΔ51 i.t. (1 × 10 8 p.f.u.) and/or colchicine i.p. (1.5 mg kg −1 ). Tumour sizes were measured every other day using an electronic caliper. Ovarian cancer model ( Fig. 2c ), T-Antigen-positive tgMISIIR-TAg (Tg(Amhr2-SV40TAg)1Bcv) female transgenic mice (described previously [19] ) ~10 weeks of age were treated with weekly i.p. injections of 1 × 10 8 p.f.u. VSVΔ51-GM-CSF and colchicine 1.5 mg kg −1 until end point as determined by the animal care guidelines. Doses were adjusted to body weights of individual mice to account for weight gain over time. All experiments were performed in accordance with the University of Ottawa Animal Care and Veterinary Services guidelines for animal care under the protocol OGHRI-58. A minimum of three mice per group was considered sufficient to detect a significant difference in tumour size over time, whereas six or more mice were considered necessary to detect a meaningful difference in survival. Microarrays and analysis 786-O cells were plated at a density of 4 × 10 5 cells in six-well flat bottom plate (Costar). Following overnight growth, cells were treated with 100 nM colchicine or vehicle. Following a 4-h pretreatment, PBS or VSVΔ51 at an MOI of 0.01 was added to cell cultures. Twenty-four hours post infection, RNA was collected using an RNA-easy kit (Qiagen, Valencia, CA, USA). RNA quality was measured using Agilent 2100 Bioanalyzer (Agilent Technologies) before hybridization. Biological triplicates were subsequently pooled and hybridized to Affymetrix human gene 1.0 ST arrays. Microarray data were processed using AltAnalyze v2.0 under default parameters [45] . A detection above background score >70 and a pV<0.05 were used to filter probe sets. By subsequently evaluating gene expression using constitutive probe sets shared across splice variants, our analysis focused on changes in gene transcription rates rather than alternative splicing mechanisms. Gene enrichment analyses were subsequently focused on 248 genes induced or repressed twofold by VSVΔ51 relative to all other data sets ( Z -test P <0.05, Benjamini–Hochberg correction). Gene ontology (GO)-term enrichments were evaluated using GOrilla [21] following correction for multiple hypothesis testing (Bonferonni). Pathway enrichments were evaluated using David following correction for multiple hypothesis testing (Benjamini–Hochberg). Raw and processed microarray data have been deposited in the ArrayExpress database E-MTAB-2433. Cell lysis and western blotting Whole-cell extracts were obtained by lysing in 50 mM HEPES, pH 7.4, 150 mM NaCl, 10 mM EDTA, 10 mM Na 4 P 2 O 7 , 100 mM NaF, 2 mM Na 3 VO 4 , protease inhibitor cocktail (Roche) and 1% Triton X-100 as described [46] . Following protein determination by Bradford assay (Bio-Rad Protein Assay Solution, Mississauga, ON), 10–20 μg of clarified cell extract were electrophoresed on 4–12% precast gradient gels (Invitrogen) using the NuPAGE SDS–PAGE Gel system (Invitrogen) with 2-(N-morpholino) ethanesulfonic acid (MES) running buffer and transferred on nitrocellulose membranes (Hybond-C, Bio-Rad). Blots were blocked with 5% nonfat milk and probed with rabbit polyclonal antibodies specific for VSV (a gift from Dr Earl Brown, used at 1:5,000 overnight), or IFNβ (sc-20107, Santa Cruz Biotechnology, Dallas, TX, used at 1:500 overnight), with GAPDH (ab37168, Abcam, Cambridge, UK, used at 1:10,000) as a loading control, followed by horseradish peroxidase-conjugated rabbit or mouse secondary antibodies, respectively (Jackson ImmunoResearch Laboratories, West Grove, PA). Membranes were washed with Tris-buffered Saline with Tween. Bands were visualized using the Supersignal West Pico Chemiluminescent substrate (Thermo Scientific Pierce, Rockford IL). Images have been cropped for presentation and full-sized images are presented in Supplementary Fig. 12a,e . Nuclear/cytoplasmic fractionation and western blotting Cell fractionation experiments were performed as previously described [46] . Briefly, cells were washed with ice-cold PBS, swelled in Hypotonic buffer (0.5 M HEPES pH 7.9, 0.1 M EGTA, 0.1 M EDTA with protease and phosphatase inhibitors), lysed with 0.1% NP-40 and cytoplasmic fractions collected using low-speed centrifugation. Nuclear proteins were then extracted with hypertonic buffer (0.5 M HEPES pH 7.9, 2.5 M NaCl, 0.1 M EGTA, 0.1 M EDTA, 30% glycerol, 20 mM NaF, 1 mM Na 3 VO 4 , 1 mM Na 4 P 2 O 7 , 1 mM dithiothreitol (DTT) and protease inhibitor cocktail) and clarified. Nuclear and cytoplasmic fractions were resolved using gel electrophoresis as above and membranes blocked with 5% BSA, cut into strips and probed for the tyrosine-701 phosphorylated (that is, activated) form of Stat-1 (9171S, Cell Signaling/New England Biolabs, Whitby, ON, 1:1,000 overnight), total Stat-1 (9172S, NEB, 1:1,000 overnight), serine-396-phosphorylated IRF-3 (4947S, NEB, 1:1,000 overnight) or total IRF-3 (FL425 SC-9082, Santa Cruz Biotechnology, 1:1,000 overnight). Antibodies against α-tubulin (sc-8035, Santa Cruz Biotechnology, 1:500 overnight) and β-actin (4970S, NEB, 1:1,000 overnight) were used as loading controls. Images have been cropped for presentation and full-sized images are presented in Supplementary Fig. 12b–d . Quantitative real-time PCR 786-0 cells were pretreated for 4 h with 0.1 μM colchicine or DMSO, and were infected with VSVΔ51 at MOI 0.01 or mock. Sixteen hours later, cells were collected and fractionated in nuclear and cytoplasmic fractions (Norgen Biotek Corp, ON, Canada). RNA extraction was performed using Qiagen QiaShredder columns and the Qiagen RNeasy kit (Qiagen). RNA (2 μg) was converted to cDNA with Superscript II Reverse Transcriptase (Invitrogen). Real-time PCR reactions were performed with the QuantiTect SYBR Green PCR kit (Qiagen) on a Rotor-gene RG-300 (Corbett Research, Australia). Optimal threshold and reaction efficiency were determined using the Rotor-gene software. Melt curves for each primer exhibited a single peak, indicating specific amplification, which was also confirmed by agarose gel. C t values were determined using the Rotor-gene software at the optimal threshold previously determined for each gene. Gene expression relative to GAPDH was calculated using the method described in ref. 47 . Fold induction was calculated relative to the DMSO-treated control for each gene. Primers were designed using Primer 3 v 4.0 (sequences available upon request). ELISA Cells were plated in 12-well dishes, pretreated with DMSO or 100 nM colchicine for 4 h, followed by mock infection or infection with VSVΔ51-GFP (or VSVΔ51 GM-CSF) at indicated MOI. Cell supernatants were collected at different times post infection, centrifuged to remove cellular debris and protease inhibitor cocktail aws added. ELISA was performed with the Verikine Human or Mouse IFN alpha, IFN beta or mouse GM-CSF kits as appropriate (PBL Interferon Source) by following the manufacturers’ instructions. Absorbance values at 450 nM were measured on a Multiskan Ascent Microplate Reader (MXT Lab Systems, Vienna, VA). Polysome profiling Cells were cultured in 15-cm dishes until confluent monolayers were formed and then pretreated with colchicine (100 nM) or vehicle (DMSO) for 4 h followed by infection with VSV at 0.1 MOI. Cells were washed 24 h post infection with cold PBS containing 100 μg ml −1 cycloheximide, collected and lysed in a hypotonic lysis buffer (5 mmol l −1 Tris-HCl (pH 7.5), 2.5 mmol l −1 MgCl 2 , 1.5 mmol l −1 KCl, 100 μg ml −1 cycloheximide, 2 mmol l −1 DTT, 0.5% Triton X-100 and 0.5% sodium deoxycholate). Lysates were loaded on 10–50% sucrose density gradients (20 mmol l −1 HEPES-KOH (pH 7.6), 100 mmol l −1 KCl, 5 mmol l −1 MgCl 2 ) and centrifuged at 164,000 × g for 2 h at 4 °C. Gradients were fractionated, and the optical density (OD) at 254 nm was continuously recorded using an ISCO fractionator (Teledyne ISCO). RNA from each fraction was isolated using TRIzol (Invitrogen) and treated with DNaseTurbo (Ambion) according to the manufacturer’s instructions. Reverse transcription PCR (RT–PCR) and semiquantitative RT–PCR (qRT–PCR) reactions were carried out using SuperScript III First-Strand Synthesis System (Invitrogen) and SYBR Green Supermix (Qiagen) according to the manufacturer’s instructions using primers for human IFNβ (5′-CATTACCTGAAGGCCAAGGA-3′, 5′-CAGCATCTGCTGGTTGAAGA-3′) IFNα (5′-ACCCACAGCCTGGATAACAG-3′; 5′-ACTGGTTGCCATCAAACTCC-3′) and VSV M (5′-CGGTATTGGCAGATCAAGGT-3′; 5′-GAGCTCAATCGTTCCCTTGT-3′). Immunofluorescence and assessment of polynuclear cells Human 786-0 renal carcinoma cells, A549, A549-AT12 or normal human GM-38 lung fibroblasts were plated in 12-well dishes on glass coverslips. Following a 4-h pretreatment with 0–1 μM colchicine, or 12 nM Taxol (as indicated), wells were infected with oncolytic VSVΔ51-expressing GFP at the indicated MOIs, or were mock-infected. Alternately, cells were treated with supernatants (see below) or cytokines for experiments in Fig. 5e,g . Cells were incubated for 24 h, and subsequently fixed with 4% paraformaldehyde, quenched with 50 mM ammonium chloride, permeabilized with 0.1% triton, blocked with 1% BSA and probed for β-tubulin (1:200, ab21057, Abcam) followed by treatment with donkey anti-goat AF-594 (1:400, Invitrogen). Coverslips were mounted on slides using Prolong AntiFade with DAPI (Invitrogen) and then photographed at × 40 or × 100, as indicated, using the Zeiss Imager M1 microscope equipped with the AxioCam HRm camera (Carl Zeiss Ltd) and the Axiovision software. Polynuclear/infected cells were counted from 5–15 pictures per well (at × 40) and a minimum of 100 cells in total. Supernatant transfer and filter experiment 786-0 or GM-38 cells were cultured and plated as described above, but were instead infected with VSVΔM51-ΔG-GFP at an MOI of 10. This virus can infect cells but cannot exit the cell because of the lack of the viral G protein, thus preventing release of viral particles in the supernatant. After overnight incubation and verification of initial infection, supernatants were filtered through a 100-, 50-, 10- or 3-kDa filter (Millipore, Billerica, MA) or left unfiltered before being transferred to fresh 786-0 (or GM-38) coverslips or 96-well plates with or without 100 nM colchicine. Coverslips or 96-well plates (as indicated) were fixed, stained and polynuclear cells counted as described above. Alternately, an alamarBlue viability assay (described above) was performed. Mathematical modelling The model describing OV replication dynamics in the presence of colchicine was derived from our previous work [11] . It uses four equations describing the transition between the uninfected population (UP), the infected population (IP), the activated population (AP) and the protected population (PP) depending on the concentration of virus [V], cytotoxic cytokine [Cyt] and extracellular interferon [IFN] in the environment. These equations are: The parameters used in the above equations represent the infection rate ( K vi. ), the rate of IFN signalling activation ( K IFN on ), the rate of IFN signalling inactivation ( K IFN off ), the EC50 of IFN (EC 50 IFN ), the rate of virus-mediated cell death ( γ c ), the EC50 of the cytotoxic cytokine (EC 50 Cyt ), the rate of cytokine-mediated cell death ( γ C_Cyt )and the rate viral clearance ( K VC ). Three equations describe the concentration of virus, IFN and cytotoxic cytokine in the media. These equations are: The parameters described in the above equations represent the rate of virus budding from IP and AP ( K Bud IP and K Bud AP , respectively), the infection rate ( K vi ), the rate of virus degradation ( γ V ), the rate of internal IFN production on initial infection ( K IFN IP ), the rate of internal IFN production following activation of IFN defenses ( K IFN AP ), the rate of IFN transfer to the extracellular compartment ( K t ), the rate of IFN degradation ( γ IFN ), the rate of cytotoxic cytokine production ( K Cyt ) and the rate of cytotoxic cytokine degradation ( γ Cyt ). A Monte Carlo simulation was generated by varying the parameters in the above model within a 10-fold range ( Supplementary Table 3 ). These parameters were generated from literature-based evidence as described previously [11] . The difference between tumour and normal cells is assumed to be the values of K Bud IP and K Bud AP , which are set to be 1- to 100-fold greater in tumour cells. Simulations were performed by integrating the above equations for a population containing 2.5 × 10 5 cells in 1 ml of media infected at an MOI=0.001, calculating virus and viability at the 72-h time point for each EC 50 Cyt and K t combination, and repeating the integration 5,000 times with novel model parameters selected within the 10-fold window. All simulations were performed in Matlab using the ODE solver ode15 s under default parameters imposing a none-negativity constraint. Statistics Unless otherwise noted (see microarray analysis), analysis of variance was used to determine significance between all treatment conditions (Tukey’s post hoc test). The log-rank test was used to determine significant differences in plots for survival studies. For all studies, significance was considered to mean a P value below or equal to 0.05. Graphs and Statistics were computed using Prism 5 and Excel. Accession codes : Microarray data have been deposited in the ArrayExpress database under the accession code E-MTAB-2433 How to cite this article: Arulanandam, R. et al . Microtubule disruption synergizes with oncolytic virotherapy by inhibiting interferon translation and potentiating bystander killing. Nat. Commun. 6:6410 doi: 10.1038/ncomms7410 (2015).